Repurposing endogenous immune pathways to tailor and control chimeric antigen receptor T cell functionality Endowing chimeric antigen receptor (CAR) T cells with additional potent functionalities holds strong potential for improving their antitumor activity. However, because potency could be deleterious without control, these additional features need to be tightly regulated. Immune pathways offer a wide array of tightly regulated genes that can be repurposed to express potent functionalities in a highly controlled manner. Here, we explore this concept by repurposing TCR, CD25 and PD1, three major players of the T cell activation pathway. We insert the CAR into the TCRα gene (TRAC CAR ), and IL-12P70 into either IL2Rα or PDCD1 genes. This process results in transient, antigen concentration-dependent IL-12P70 secretion, increases TRAC CAR T cell cytotoxicity and extends survival of tumor-bearing mice. This gene network repurposing strategy can be extended to other cellular pathways, thus paving the way for generating smart CAR T cells able to integrate biological inputs and to translate them into therapeutic outputs in a highly regulated manner. Chimeric Antigen Receptor (CAR) T cell and T cell therapies hold great promise for treating a wide range of malignancies. However, these therapies face multiple challenges, including tumor accessibility, tumor-dependent inhibitory signals, and a microenvironment that is hostile to T cells. To overcome these obstacles, CAR T cells have been engineered to remove inhibitory receptors [1] , [2] , [3] , to express costimulatory molecules [3] and chemokine receptors [4] , [5] , or to secrete immunostimulatory factors such as checkpoint inhibitors [6] or cytokines [7] . In particular, cytokine secretion by so called Armored or Truck CAR T cells [7] , [8] is a highly promising strategy for improving CAR T cell function. When integrated into the T cell genome via lentiviral or gamma retroviral vector transduction, recombinant IL-12P70 [9] , [10] , [11] , [12] , IL-15 [13] , [14] , and IL-18 [15] , [16] , [17] have been reported to increase CAR T cell antitumor activity, to prevent CAR T cell anergy, to remodel the tumor microenvironment, and to recruit the innate immune cells that are necessary for the antitumor response [9] . However, as these immunostimulatory agents are highly potent, they may have side effects [18] . When secreted by CAR T cells or by Tumor Infiltrating Lymphocytes (TILs), they can generate adverse preclinical [12] , [19] and clinical [20] events, given the suboptimal control of their secretion and the high quantity of factor released in the circulation [20] , [21] . Thus, new engineering strategies that enable tight control of the production, secretion, or presentation of exogenous proteins of interest by engineered T cells will be valuable in developing the next generation of T cell-based therapies. Immune pathways, which evolved to support the survival of the host in response to infectious agents [22] , offer a wide array of tightly regulated genes that can be repurposed to secrete a protein of interest, such as a cytokine, in a conditional and highly controlled manner. For example, the activation of T cells via T cell receptor (TCR) engagement triggers a multistep signaling process that leads to the activation of transcription factors, including Nuclear Factor of Activated T cells (NFAT), which orchestrate a precise ballet of gene expression and subsequent protein translation [23] . Some of these genes, including IL-2, CD69, and IL2Rα, are rapidly induced to promote T cell proliferation, differentiation, and activation, whereas others, including PDCD1, LAG3, and FASLG, are induced later to serve as a rheostat for the immune response [24] , [25] . Thanks to transcriptional and post-translational regulation, the coordinated induction of these genes follows precise kinetics and quantitative patterns that fine-tune the functional outputs of T cells. Customizing these functional outputs by repurposing endogenous gene expression therefore represents an attractive means for generating smart CAR T cells that are able to sense and react to their environment in a tailored, highly regulated, and antigen-specific manner. We explored this concept by repurposing TCR, CD25, and PD1, three major players of the T cell activation pathway, to enable CAR T cells to secrete the pro-inflammatory cytokine IL-12P70 in a tumor cell-dependent manner. Based on the seminal work established in [26] , we use the TALEN technology with recombinant adeno-associated virus 6 (AAV6) repair vectors to place CAR and IL-12P70 expression under the control of TCR (TRAC CAR ) [26] and either IL2Rα or PDCD1 regulatory elements, respectively. This multiplex gene repurposing process leads to the expression of a CAR and to conditional secretion of IL-12P70. The secretion of IL-12P70 is transient, dependent on tumor engagement, and follows the tightly regulated patterns of CD25 and PD1 expression that are observed upon T cell activation. IL-12P70 promotes the accumulation of TRAC CAR T cells and markedly improves their antitumor activity in vitro and in vivo. Furthermore, the targeted integration of IL-12P70 at the PDCD1 locus concomitantly inactivate PD1, one of the major checkpoint of T cell function. TCR pathway repurposing via multiplex gene editing Targeted insertion via homology-directed repair is possible in primary T cells and hematopoietic stem and progenitor cells. Techniques for such insertion include AAV6 or DNA repair matrices along with site-specific engineered nucleases such as TALEN, megaTAL, meganucleases, Zinc Finger nucleases and CRISPR-CAS9 [26] , [27] , [28] , [29] , [30] , [31] , [32] , [33] , [34] , [35] . Here, we extend this approach pioneered by [26] to simultaneously engineer CAR and IL-12P70 expression under the control of TRAC and either IL2rα or PDCD1 regulatory elements (Fig. 1a ). To do so, we generated three different AAV6 promoter-less repair matrices. The first matrix, TRAC CARm , was designed to integrate an anti-CD22 CAR expression cassette at the TRAC locus [26] , [36] . This CAR architecture contains integrated purification and safeguard domains that allow purification and Rituximab-dependent depletion of TRAC CAR T cells (Supplementary Fig. 1a ) [36] . The second and third matrices, IL2rα IL12m and PDCD1 IL12m , were designed to integrate the IL-12P70 heterodimer (formed by IL-12A p35 and IL-12B p40 subunits) along with a truncated low-affinity nerve growth factor receptor (ΔLNGFR) surface marker [37] at the IL2rα and PDCD1 loci, respectively. These three matrices use the reading frame of the targeted genes and contain 2A self-cleaving elements upstream of each expression cassette and 300 bp homology arms specific for TRAC, IL2rα, or PDCD1 loci. The insertion sites for the matrices allow functional inactivation of TCR and PD1 (leading to a truncated and inactive form) and preserve the expression of CD25, an important component of the IL-2 receptor [38] , [39] (Fig. 1a ). Fig. 1 Repurposing the TCR pathway via TALEN and adeno-associated virus (AAV6) treatments. a Schematic showing the strategies used to repurpose TRAC along with the IL2rα or PDCD1 loci to generate TRAC CAR , TRAC CAR _CD25 IL12 , and TRAC CAR _ΔPD1 IL12 T cells from wild-type T cells. The genetic elements composing the TRAC and IL-12P70 matrices (TRAC CARm , IL2rα IL12m and PDCD1 IL12m ) are illustrated. TRAC CARm was designed to express a CAR architecture via the TRAC locus, and IL2rα IL12m and PDCD1 IL12m were designed to express IL-12P70 and ΔLNGFR via the IL2rα and PDCD1 loci. The three matrices keep the reading frame of the targeted genes, and they contain 2A self-cleaving elements upstream of each expression cassette and 300-bp homology arms that are specific for each locus. The matrix insertion locations were chosen to inactivate TCR and PD1 (expression of truncated/inactive form after insertion) and to preserve CD25 expression. b Experimental design for multiplex repurposing of TRAC, IL2rα or PDCD1 and analysis of the resulting engineered TRAC CAR T cells. c and d Frequency of TCRαβ (−) T cells and of TCRαβ (−) CAR (+) T cell observed by flow cytometry, respectively, 6 days post TALEN mRNA electroporation and AAV6 transduction. Each point represents one experiment performed with a given donor. n = 11 for TRAC CAR , n = 7 for TRAC CAR _CD25 IL12 and n = 7 for TRAC CAR _ΔPD1 IL12 T cells. One-way ANOVA was used in panel d for statistical analysis (ns not significant). e – g Summary of engineered TRAC CAR T cell production. TRAC CAR T cells generated from 3 independent donors were analyzed at the end of their production. e , f , and g show the number of TRAC CAR T cells obtained at the end of a GREX10 culture, the frequency of viable cells, and the quantity of IL-12P70 detected in the culture supernatants (Lower limit of IL12P70 detection 9.8 pg/mL), respectively. Each point represents one experiment performed with a given donor. n = 3 for each engineered TRAC CAR T cells batch. On each box plot, the central mark indicates the median, the bottom and top edges of the box indicate the interquartile range (IQR) and the whiskers represent the maximum and minimum data points. Source data are provided as a Source Data file Full size image To demonstrate that CAR and IL-12P70 expression can be placed under the control of the TRAC and IL2rα or PDCD1 regulatory elements, respectively, we simultaneously transduced T cells with TRAC CARm and either IL2rα IL12m or PDCD1 IL12m after TALEN treatment (Fig. 1b ) to generate TRAC CAR _CD25 IL12 , or TRAC CAR _ΔPD1 IL12 T cells, respectively (Fig. 1a ). Reference controls consisted in treating only with TRAC TALEN and TRAC CARm repair template (named TRAC CAR cells), or by simply omitting the IL-12 repair matrix while maintaining double TALEN treatment and CAR transduction (TRAC CAR _CD25 and TRAC CAR _ΔPD1 T cells), were generated to account for the effect of IL2Rα or PDCD1 TALEN independently of IL-12. We observed efficient TCR knockout (>90% TCRαβ (−) T cells, Fig. 1c ) and targeted expression of CAR at the TRAC locus (up to 65% of CAR (+) TCRαβ (−) T cells, Fig. 1d ) 6 days after treatment. Similar results were obtained under the three different conditions, indicating that the presence of multiple TALEN constructs and the IL-12P70 repair matrix do not disturb the targeted CAR insertion at the TRAC locus. This engineering process did not affect the viability or the proliferation capacity of TRAC CAR T cells (Fig. 1e, f ) and led to low levels of IL-12P70 secretion in the culture media after 15 days of expansion (lower level of detection was determined at 9.8 pg/mL). Furthermore, it did not affect our ability to purify and efficiently deplete TRAC CAR T cells with the FDA-approved drug Rituximab (RTX), as demonstrated previously using a lentiviral-based vectorization approach (Supplementary Figs. 1 and 2 [36] ). Specificity of TCR pathway repurposing Targeted insertion of the three matrices was confirmed using Targeted Locus Amplification (TLA), a method enabling genome wide, unbiased mapping of transgene insertion [40] (Fig. 2 ). As expected, TRAC CARm , IL2rα IL12m and PDCD1 IL12m were specifically inserted into chromosome 14, 10, or 2 respectively (Fig. 2a, c ). The majority of transgenes were inserted in frame with the intended open reading frame. We also found low coverage of TRAC CARm on chromosome 10 or 2 (PDCD1 and IL2rα loci) and of IL2rα IL12m or PDCD1 IL12m on chromosome 14 (TRAC Locus). The molecular signature of these marginal events suggests co-integration of matrices concatemeres at TRAC, IL2rα, and PDCD1 loci in a few cells, although we cannot exclude homology-independent trapping of matrices at the three loci. Fig. 2 Cytogenetic and genomic characterization of engineered TRAC CAR T cells. a Targeted locus amplification (TLA) analysis of TRAC CAR _ΔPD1 IL12 cells using TRAC CARm specific primers (left panel) or PDCD1 IL12m specific primers (right panel). Specific targeted integration coverages and potential concatemere or homology-independent integrations are indicated by red and blue boxes, respectively. b , left panel Frequency of translocation events between TRAC and PDCD1 loci detected by FISH in MRC5 standard cell line ( n = 100 metaphases analyzed) and in TRAC CAR _ΔPD1 IL12 ( n = 500 metaphases analyzed). Cells harboring or not the expected gene fusion named 14q11.2_2q37 are illustrated in red or black, respectively and the number of metaphase analyzed for each sample are indicated. b , right panel Representative example of TRAC CAR _ΔPD1 IL12 cells karyotype showing normal ploidy level and no sign of genetic alteraction of TRAC and PDCD1 chromosomal loci. c Targeted locus amplification analysis of TRAC CAR _CD25 IL12 cells using TRAC CARm specific primers (left panel) or IL2rα IL12m specific primers (right panel). Specific targeted integration coverages and potential concatemere integrations are indicated by red and blue boxes, respectively. d , left panel Frequency of translocation events between TRAC and IL2rα loci detected by FISH in MRC5 standard cell line ( n = 100 metaphases analyzed) and in TRAC CAR _CD25 IL12 ( n = 500 metaphases analyzed). Cells harboring or not the expected gene fusion named 14q11.2/10p15.1 are indicated in red and black, respectively and the number of metaphase analyzed for each sample are indicated. Chi square was used to calculate the statistical significance of FISH analysis. d , right panel Representative example of TRAC CAR _CD25 IL12 karyotype showing normal ploidy and no sign of genetic alteration of IL2rα and TRAC chromosomal loci. The TLA and FISH plots and Karyotype figures represents 1 experiment performed with 1 donor. Source data are provided as a Source Data file Full size image Because simultaneous TALEN treatment could lead to unwanted genetic adverse events including translocation between two targeted loci [41] , [42] , we characterized cytogenic properties of engineered TRAC CAR _CD25 IL12 and TRAC CAR _ΔPD1 IL12 T cells thoroughly by karyotyping and Fluorescence-In-Situ-Hybridization (FISH). Karyotyping and G-banding pattern results were consistent with human diploid samples devoid of gross structural abnormalities or clonal chromosomal aberrations (Fig. 2b, d ). Consistently, FISH analysis did not show significant difference ( p = 0.766, Chi square) between the frequency of TRAC/PDCD1 or TRAC/IL2Rα gene fusion obtained in engineered T cells and in MRC5, a human fibroblast cell line considered a reference diploid cell line and commonly used as a negative control for gene fusion detection (Fig. 2b, d ). Although the low sensitivity of this test does not rule out translocation (sensitivity of FISH analysis ~ 1–4%), it indicated that they were not markedly enriched over the standard expansion process used to produce TRAC CAR T cells. Further work will be needed to thoroughly address this point before moving toward clinical applications. Disruptive and non disruptive targeted insertion of IL-12P70 After demonstrating targeted insertion of the three matrices, we verified that the delivery of PDCD1-specific and IL2rα-specific TALEN disrupted PD1 and spared CD25 surface presentation in the presence or absence of appropriate IL-12P70 repair matrices. After activation of engineered TRAC CAR T cells with RAJI cells (E/T = 1) and T cell analysis by flow cytometry to determine CD25 and PD1 expression (Fig. 3a ), we observed similar frequencies of CD25 expression among the three different conditions (Fig. 3b ). This indicated that TALEN-mediated processing of the 3’UTR of IL2rα gene (Supplementary Fig. 3a ) did not impair CD25 surface expression. In contrast, PD1 expression was significantly impaired, as illustrated by the difference between the surface expression of PD1 in the PDCD1 TALEN-treated TRAC CAR T cells (TRAC CAR _ΔPD1 and TRAC CAR _ΔPD1 IL12 T cells) and that of the TRAC CAR T cell control (Fig. 3c , one way Anova, p < 0.0001 for both comparisons). Consistently, high throughput DNA sequencing showed that PDCD1 TALEN treatment promoted 66% of indels at the PDCD1 locus (Supplementary Fig. 3a ). Because of its potential for downstream clinical application, we further characterized the specificity of TRAC/PDCD1 TALEN co-treatment using an Oligo capture assay derived from ref. [43] and high throughput DNA sequencing (Supplementary Fig. 3b ). The potential offsite candidates identified in T cells treated with TRAC and PD1 TALEN showed similar frequency of insertion and deletions (Indels) than the ones detected in mock-treated T cells. Thus, TRAC/PDCD1 TALEN co-treatment did not lead to offsite targeting above the natural mutation rate observed in primary T cells. Fig. 3 Efficient translation of tumor cell engagement by TRAC CAR T cell into IL-12P70 secretion in vitro. a Schematic showing the experimental design used to determine the levels of CD25 and PD1 expression and IL-12P70 secretion by tumor cell-activated TRAC CAR T cells. b and c Frequency of CD25 and PD1 expression detected among TCRαβ (−) and CAR (+) T cells, respectively. Each point represents one experiment performed with a given donor ( n = 7). One-way ANOVA was used in panel 3b and 3c for statistical analysis and p -value are indicated. d Schematic showing the expected outcome of IL-12P70 secretion upon tumor cell engagement by TRAC CAR _CD25 or TRAC CAR _CD25 IL12 T cells. e Flow cytometry plots showing ΔLNGFR surface expression 48 h after tumor cell-dependent activation of TRAC CAR _CD25 and TRAC CAR _CD25 IL12 T cells. The flow plot was obtained using engineered TRAC CAR T cell batches harboring the highest IL-12P70 targeted integration. The red box indicates the proportion of ∆LNGFR expressed by successfully engineered TRAC CAR T cells. Gating strategy is illustrated in Supplementary Fig. 4 . f Schematic showing IL-12P70 secretion upon tumor cell engagement by TRAC CAR _ΔPD1 or TRAC CAR _ΔPD1 IL12 T cells. g Flow cytometry plots showing the level of ΔLNGFR expression, 48 h after tumor cell-dependent activation of TRAC CAR _CD25 and TRAC CAR _CD25 IL12 T cells. The solid blue squares indicate the frequency of ∆LNGFR expression by successfully engineered TRAC CAR T cells. Gating strategy is illustrated in Supplementary Fig. 4 . h Frequency of ∆LNGFR expression (left panel) and quantity of IL-12P70 secreted (right panel) by TRAC CAR T cells engineered at the IL2rα and PDCD1 loci, 48 h after tumor cell-dependent activation of the TRAC CAR T cells. Each point represents one experiment performed with a given donor ( n = 6) and the threshold of IL-12P70 detection is 5 pg/mL. On each box plot, the central mark indicates the median, the bottom and top edges of the box indicate the interquartile range (IQR) and the whiskers represent the maximum and minimum data point. One-way ANOVA was used in panel 3h for statistical analysis and p -value are indicated. Source data are provided as a Source Data file Full size image Translating tumor cell engagement into secretion of IL-12P70 We indirectly determined the efficiency of IL-12P70 matrix insertion at the IL2rα or PDCD1 loci by assessing the expression of ΔLNGFR at the surface of TRAC CAR T cells and characterizing IL-12P70 secretion upon tumor cell engagement. For this purpose, we activated TRAC CAR T cells with RAJI cells as described above (Fig. 3a ) and then analyzed T cells using flow cytometry. We observed an increase in ΔLNGFR expression in TRAC CAR T cells engineered to express IL-12P70 under the control of IL2rα regulatory elements (Fig. 3e , red square). Consistently, ΔLNGFR was only detected in CD25 (+) TRAC CAR T cells, suggesting an efficient targeted insertion of the IL-12P70 matrix at the IL2rα locus. Similar results were obtained with TRAC CAR T cells engineered to express IL-12P70 under the control of PDCD1 regulatory elements, in which we also observed an increase of ΔLNGFR upon tumor cell engagement (Fig. 3g , blue square). However, in contrast to the IL2rα locus, the majority of ΔLNGFR-positive cells were PD1-negative, as expected for a matrix designed to interrupt the PDCD1 coding sequence. A significant increase of ΔLNGFR expression by TRAC CAR _CD25 IL12 T cells compared to TRAC CAR _CD25 T cells ( p = 0.034, one-way ANOVA) and a marked increase of ΔLNGFR expression by TRAC CAR _ΔPD1 IL12 T cells compared to TRAC CAR _ΔPD1 T cells was observed for multiple T cell donors engineered to target the IL2rα and PDCD1 loci (Fig. 3h ). To determine whether there was a correlation between the tumor cell-dependent expression of ΔLNGFR by TRAC CAR T cells and IL-12P70 secretion, we characterized the supernatants recovered after two days of TRAC CAR T cell/tumor cell co-culture through ELISA quantification (Fig. 3a and Fig. 3h right panel). TRAC CAR T cells secreted medians of 23 or 49 pg of IL-12P70/mL/12 h when the IL-12P70 matrix was inserted at the PDCD1 locus or the IL2rα locus, respectively. In contrast, TRAC CAR T cells lacking IL-12P70m secreted significantly less IL-12P70 (one way Anova, p = 0.023 and p < 0.0001 for PDCD1 and the IL2rα locus, respectively) showing levels of secreted IL-12P70 lying within the threshold of detection (5 pg/mL). These results indicate that IL2rα or PDCD1 can be rewired to secrete IL-12P70 in a tumor cell-dependent manner. Secretion of IL-12P70 by TRAC CAR T cell is tighly regulated To explore the temporal regulation of IL-12P70 in response to tumor cell engagement, we characterized the kinetics of CD25, PD1, and ΔLNGFR expression upon repeated stimulations with tumor cells. To this end, we cultured TRAC CAR T cells with tumor cells on days 0 and 4 and monitored surface protein expression by flow cytometry (Fig. 4 ). We observed a biphasic pattern of PD1 and CD25 expression after tumor cell engagement by TRAC CAR T cells (Fig. 4a , top panels). This trend, reproduced after the second tumor cell engagement, indicates that the expression of both proteins is tightly upregulated and downregulated upon CAR activation. This regulation was also observed for ΔLNGFR expression and IL-12P70 secretion, demonstrating that the ΔLNGFR and IL-12P70 transgenes benefited from the IL2rα and PDCD1 endogenous regulatory elements (Fig. 4a ). Notably, ΔLNGFR and IL-12P70 were induced faster than CD25 after the first tumor cell engagement, suggesting that there are differences in the trafficking or cell surface multimerization kinetics between these proteins. In addition, while the downregulation of CD25 and PD1 led to an almost complete shutdown of their expression, this phenomenon showed subtle kinetic differences that paralleled ΔLNGFR expression and IL-12P70 secretion levels. Indeed, PD1 expression was still detectable at day 3, when CD25 expression reached its basal level. This difference was also observed for the corresponding ΔLNGFR surrogate and for IL-12P70, found to be secreted over a longer time by TRAC CAR _ΔPD1 IL12m than by TRAC CAR _CD25 IL12m . Similar results were obtained when IL-15/IL-15rα was substituted for IL-12P70, demonstrating the robustness and transposability of our approach to express proteins of therapeutic interest [44] , [45] in a tumor cell-dependent manner (Supplementary Fig. 4 ). Fig. 4 The secretion of IL-12P70 by TRAC CAR T cells is regulated by tumor cell engagement in vitro. a Kinetics of CD25 and PD1 expression (top), ΔLNGFR expression (middle), and IL-12P70 secretion (bottom panel) in purified TRAC CAR T cells after two consecutive tumor cells challenges. TRAC CAR T cells were activated by RAJI cells at day 0 and day 4 and analyzed by flow cytometry for 8 days. IL-12P70 secreted in cell culture supernatants was quantified by ELISA and plotted as a function of time. The arrows indicate the times of tumor cell addition. The data shown represent the average +/− standard deviation of two experiments performed with cells from two different donors. b Changes in ΔLNGFR reporter expression and IL-12P70 secretion as a function of tumor cell concentration. Engineered TRAC CAR T cells were activated by different quantities of RAJI cells for 48 h. Supernatants were used to quantify IL-12P70 via ELISA assays and cells were analyzed by flow cytometry to evaluate the frequency of ΔLNGFR+ cells, as well as its mean fluorescence intensity. Values are plotted as a function of the tumor cell to TRAC CAR T cell ratio. The data shown are the average +/− standard deviation of three experiments performed with cells from three different donors. Source data are provided as a Source Data file Full size image We benchmarked our repurposing strategy to the engineering approach developed earlier to reexpress IL-12P70 [20] , [21] , [46] , [47] in a tumor cell-dependent manner. To do so, we first assessed the level of IL-12P70 secreted by T cell transduced with increasing amounts of rLV particles encoding NFAT IL-12P70, a construct previously designed to express an IL-12P70 under the control of 6xNFAT promoter [20] , [21] . Transduced cells obtained from one donor were co-cultivated with and without PMA ionomycin to determine the basal and activation-dependent levels of IL-12P70 secretion. Consistent with former studies [21] , [48] , IL-12P70 was efficiently secreted upon activation, but also detected in the absence of activation indicating a suboptimal control of secretion. To confirm this aspect, we compared the levels of IL12P70 secretion by TRAC CAR _ΔPD1 IL12 and by CAR T cell transduced with low MOI of NFAT IL-12P70 rLV particle (CAR_NFAT IL12 , MOI = 0.25) before, during, and after tumor cell engagement (Supplementary Fig. 6d ). Our results showed that both engineering strategies enable tumor-cell-dependent secretion of IL-12P70. However, CAR_NFAT IL12 displayed basal leakiness, as illustrated by the presence of substantial levels of IL-12P70 before and after 8 days of tumor cell challenge (Supplementary Fig. 6d ). This pattern contrasted with the one obtained from TRAC CAR _ΔPD1 IL12 cells, consistently showing low secretion of IL-12P70 before and after 8 days of tumor cell challenge. To characterize the control of gene expression after tumor cell engagement further, we assessed if an increased tumor cell concentration correlated with the level of IL-12P70 secretion by TRAC CAR T cells. To do so, we incubated TRAC CAR T cells in the presence of increasing concentration of tumor cells for two days and measured the levels of secreted IL-12P70 (Fig. 4b ). The extent of IL-12P70 secretion increased as a function of tumor cell concentration and reached a plateau at a tumor-to-TRAC CAR T cell ratio of 1-to-1 (Fig. 4b ). Interestingly, the repurposed IL2rα locus elicited a higher maximum level of IL-12P70 secretion than the PDCD1 locus. This correlated with the significant differences observed between the quantity of IL-12P70 secreted by PDCD1 and IL2rα loci (Fig. 3h right, p ≤ 0.023, one-way ANOVA) and suggests that the level of therapeutic product secretion could be controlled by careful selection of a locus to repurpose. Tumor-dependant and local delivery of IL-12P70 in vivo As the IL2rα and PDCD1 loci can be efficiently repurposed to secrete IL-12P70 in a controlled and tumor-dependent manner in vitro, we tested whether the IL-12P70 secreting TRAC CAR T cells could transiently and locally deliver IL-12P70 to an engrafted tumor in a xenogenic mouse model. For that purpose, CD22(+) and CD22(−) RAJI tumor cells expressing firefly luciferase were transplanted subcutaneously into the left and right flanks of NSG mice, respectively (Fig. 5a ). Mice were then randomized on the basis of their luminescence signal three days after transplantation and injected intravenously with TRAC CAR _CD25, TRAC CAR _CD25 IL12 , TRAC CAR _ΔPD1, or TRAC CAR _ΔPD1 IL12 T cells. Four days after TRAC CAR T cell transfer, the tumors were analyzed by flow cytometry and ELISA. TRAC CAR T cells were robustly detected at the CD22(+) tumor site (left flank) but were almost absent from the CD22(-) tumor site (right flank, Fig. 5b , left graph), indicating that TRAC CAR T cells preferentially accumulate at their intended tumor-specific site. The frequencies of TRAC CAR T cells detected at the CD22(+) tumor sites were similar in all groups regardless of IL-12P70 status (Fig. 5b , left graph), suggesting that genetic engineering does not affect the trafficking or early accumulation of T cells. IL-12P70 secretion was significantly lower in the CD22(−) right tumor site than in the CD22(+) left tumor site (Fig. 5c , Wilcoxon-Mann-Whitney test, p = 0.018 and 0.03 for TRAC CAR _CD25 IL12 and TRAC CAR _ΔPD1 IL12 , respectively), suggesting that IL-12P70 can be conditionally and locally delivered to a specific tumor site in vivo by TRAC CAR T cells. Fig. 5 In vivo local and tumor-dependent delivery of IL-12P70 by TRAC CAR T cells. a Schematic showing the experimental design to study the tumor-dependent secretion of IL-12P70 by TRAC CAR T cells in NSG mice (BLI: bioluminescence). CD22(+) and CD22(−) RAJI tumor cells expressing firefly luciferase were transferred subcutaneously into the left (L) and right (R) flanks of NSG mice, respectively, and allowed to engraft for 4 days before TRAC CAR T cell transfer. Four days after TRAC CAR T cells transfer, tumors and T cells were recovered, dissociated, and analyzed via flow cytometry and ELISA. b Frequency of TRAC CAR T cells detected by flow cytometry at the left (L) and right (R) flanks of NSG mice. A non parametric paired Mann-Whitney test was used for statistical analysis of the data ( p -value are indicated). c Quantity of IL-12P70 detected in the left (L) and right (R) flanks of NSG mice. Each point documented in b and c represents the result obtained in each mice ( n = 4 for TRAC CAR _CD25, n = 6 for TRAC CAR _CD25 IL12 , n = 3 for TRAC CAR _ΔPD1, n = 5 for TRAC CAR _ΔPD1 IL12 ). On each box plot, the central mark indicates the median, the bottom and top edges of the box indicate the interquartile range (IQR) and the whiskers represent the maximum and minimum data point. A paired Wilcoxon-Mann-Whitney non-parametric test was used for statistical analysis of the IL-12P70 quantities obtained at the right and left flanks of the same animal (p-value are indicated). Source data are provided as a Source Data file Full size image Secretion of IL-12P70 improves TRAC CAR T cells activity As the secretion of IL-12P70 by TILs and CAR T cells can enhance the cytolytic properties of CAR T cells in vitro and in vivo [9] , [20] , [21] , [49] , we asked whether the amount of IL-12P70 secretion observed during TRAC CAR T cell activation in vitro (Fig. 4 ) was sufficient to improve antitumor activity. To test this, we compared in vitro the short-term and long-term antitumor activities of purified TRAC CAR T cells (100% CAR positive T cells) with or without transgenic IL-12P70 expression. Short-term antitumor activity was characterized in vitro by using the activation protocol described in Fig. 3a (between days 10 and 12) and kinetics of tumor cell disappearance were monitored by flow cytometry. After the first tumor cell challenge, IL-12P70-expressing TRAC CAR T cells elicited a faster tumor cell clearance than control TRAC CAR T cells (Fig. 6a ; Supplementary Fig. 7 ). This kinetic difference, also observed after the second tumor cell challenge, resulted in more than a 100-fold difference in residual tumor cells detected after 8 days of culture with and without IL-12P70. Thus, we hypothesized that the IL-12P70-mediated increase in tumor cell clearance rate might translate into long-term tumor cell control by TRAC CAR T cells, even after repeated tumor cell challenges. We performed an in vitro serial killing assay [36] that allowed us to repeatedly challenge TRAC CAR T cells with daily doses of tumor cells for 8 consecutive days (Fig. 6b ). To ensure efficient discrimination between the activity of IL-12P70-secreting TRAC CAR T cells and control TRAC CAR T cells, the daily doses of tumor cell were increased 5-fold (from 1× to 5×) during the last 4 days of this assay. Daily challenges of TRAC CAR T cells edited by either IL2rα or PDCD1 TALEN in the absence of the IL-12P70 matrix (TRAC CAR _CD25 and TRAC CAR ΔPD1, black open circles, Fig. 6b ) resulted in suboptimal tumor cell control and eventual tumor cell outgrowth. In contrast, IL-12P70-secreting TRAC CAR T cells (TRAC CAR _CD25 IL12 , red open circles, and TRAC CAR _ ΔPD1 IL12 , blue open circles, Fig. 6b , upper panel) showed continuous and efficient tumor cell control correlated with the secretion of IL-12P70 and increased surface expression of CD62L (Fig. 6c, d ). In the same in vitro assay, IL-12P70 secretion significantly improved the expansion of CD8+ TRAC CAR T cells (Fig. 6b lower panel, p = 0024 and p = 0.052 for TRAC CAR _CD25 IL12 and TRAC CAR _ΔPD1 IL12 , respectively). In addition, we compared the cytotoxic activity of rLV CAR_NFAT IL12 and AAV6-based TRAC CAR _ΔPD1 IL12 engineered CAR T cells (Supplementary Figs. 6e and 5f ) using a similar serial killing assay. Both engineering strategies led to similar cytotoxic activity and confirmed the immunostimulatory effect of IL-12P70 on CAR T cell antitumor activity. Fig. 6 Conditional secretion of IL-12P70 increases TRAC CAR T cells antitumor activity in vitro. a Kinetics of tumor cell clearance by purified TRAC CAR T cells and TRAC CAR T cells secreting IL-12P70. TRAC CAR , TRAC CAR _CD25 IL12 T cells and TRAC CAR _ΔPD1 IL12 T cells were challenged with 1 equivalent of RAJI cells at days 0 and 4 and cultivated for 8 days. Kinetics of tumor cell disappearance was analyzed by integrating flow cytometry data, using CD19 antibody specific for RAJI cells, and total number of cells mixture. The relative tumor cell count was computed as the ratio of remaining tumor cells at a given time to the total number of tumor cells added. b Long-term cytotoxicity assay. TRAC CAR T cells were challenged daily with RAJI cells at a ratio of T cells to tumor cells of 5-to-1. Fresh tumor cells (0.2 × 10 6 cells) were added everyday up to day 4 after pelleting and resuspended the TRAC CAR T cells in fresh culture media. From day 5 onward, 5× the original number of tumor cells (10 6 cells) was added. The antitumor activity of the TRAC CAR T cells was monitored everyday by measuring the luminescence of the remaining RAJI tumor cells expressing luciferase. Cells were counted and analyzed by flow cytometry on days 0, 2, 5, and 8, and the number of CD8 (+) CAR T cells was computed and plotted as a function of time. The data are averaged +/− standard deviation from two experiments performed with cells from two different donors. Two-way ANOVA was used in panel b for statistical analysis ( p -value are indicated). c Comparison of IL-12P70 secretion for different TRAC CAR T cell groups at day 5 of the serial killing assay. d Comparison of CD62L MFI among CD8 (+) CAR T cells obtained for the different TRAC CAR T cell groups at day 8 of the serial killing assay. The data shown in c and d were obtained from two experiments performed with cells from two different donors. On each box plot, the central mark indicates the median, the bottom and top edges of the box indicate the interquartile range and the whiskers represent the maximum and minimum data point. Source data are provided as a Source Data file Full size image In previous studies [11] , [50] , [51] , the presence of IL-12P70 at the time of T cell activation was reported to simultaneously support increased CD62L expression and enhanced effector function. To investigate this aspect in more details, we performed cytokine and surface marker profiling of TRAC CAR T cells chronically challenged by RAJI cells for four days of cell culture (Fig. 7a ). Comparison of CD62L and CD45RA surface markers expression indicated that IL-12P70 expressing TRAC CAR T cells retained a higher frequency of naïve markers and a lower frequency of effector markers than their TRAC CAR T cell counterparts (Fig. 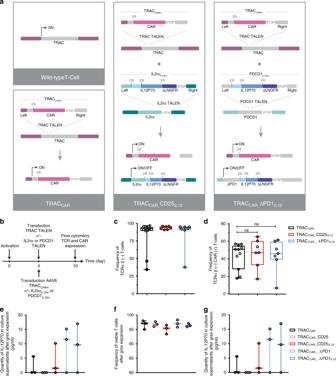Fig. 1 Repurposing the TCR pathway via TALEN and adeno-associated virus (AAV6) treatments.aSchematic showing the strategies used to repurpose TRAC along with the IL2rα or PDCD1 loci to generate TRACCAR, TRACCAR_CD25IL12, and TRACCAR_ΔPD1IL12T cells from wild-type T cells. The genetic elements composing the TRAC and IL-12P70 matrices (TRACCARm, IL2rαIL12mand PDCD1IL12m) are illustrated. TRACCARmwas designed to express a CAR architecture via the TRAC locus, and IL2rαIL12mand PDCD1IL12mwere designed to express IL-12P70 and ΔLNGFR via the IL2rα and PDCD1 loci. The three matrices keep the reading frame of the targeted genes, and they contain 2A self-cleaving elements upstream of each expression cassette and 300-bp homology arms that are specific for each locus. The matrix insertion locations were chosen to inactivate TCR and PD1 (expression of truncated/inactive form after insertion) and to preserve CD25 expression.bExperimental design for multiplex repurposing of TRAC, IL2rα or PDCD1 and analysis of the resulting engineered TRACCART cells.canddFrequency of TCRαβ (−) T cells and of TCRαβ (−) CAR (+) T cell observed by flow cytometry, respectively, 6 days post TALEN mRNA electroporation and AAV6 transduction. Each point represents one experiment performed with a given donor.n= 11 for TRACCAR,n= 7 for TRACCAR_CD25IL12andn= 7 for TRACCAR_ΔPD1IL12T cells. One-way ANOVA was used in paneldfor statistical analysis (ns not significant).e–gSummary of engineered TRACCART cell production. TRACCART cells generated from 3 independent donors were analyzed at the end of their production.e,f, andgshow the number of TRACCART cells obtained at the end of a GREX10 culture, the frequency of viable cells, and the quantity of IL-12P70 detected in the culture supernatants (Lower limit of IL12P70 detection 9.8 pg/mL), respectively. Each point represents one experiment performed with a given donor.n= 3 for each engineered TRACCART cells batch. On each box plot, the central mark indicates the median, the bottom and top edges of the box indicate the interquartile range (IQR) and the whiskers represent the maximum and minimum data points. Source data are provided as a Source Data file 7b and Supplementary Table 1 ). Consistent with earlier reports [52] , this phenomenon was correlated with a significant increase of IL-2 ( p < 0.0001 for TRAC CAR _CD25 IL12 and TRAC CAR _ΔPD1 IL12 , two-way ANOVA), TNFα ( p = 0.0013 for TRAC CAR _CD25 IL12 , two-way ANOVA) for and IL-10 secretion ( p < 0.02 for TRAC CAR _CD25 IL12 and TRAC CAR _ΔPD1 IL12 , two-way ANOVA) and a marked increase of IFNγ secretion by engineered cells (Fig. 7c ). Interestingly, IL-12P70 secretion correlated with a significant increase of IL-4 ( p < 0.05, for TRAC CAR _CD25 IL12 and TRAC CAR _ΔPD1 IL12 , two-way ANOVA), although the fold change was negligible. In addition, IL-5 was markedly, although not significantly, decreased in IL-12P70 secreting TRAC CAR T cells groups. Fig. 7 Immunoprofiling of engineered TRAC CAR T cells activated by tumor cells in vitro. a Schematic showing the experimental design to investigate the effector and memory phenotype and cytokine secretion profile of activated engineered TRAC CAR T cells. 10 6 TRAC CAR T cells were mixed with a suspension of RAJI-luc tumor cells at E:T = 5:1 in a total volume of 40 mL of Xvivo-15 media supplemented with 5% AB serum and incubated in a GREX-10 device. The mixture was incubated for 24 h before adding 2 × 10 6 RAJI-Luc cells. The resulting cell mixture was incubated for 24 h and the same procedure was repeated to get a total of 4 RAJI cell challenges. The mixture was then incubated as is for 4 additional days and where spun down to recover the supernatant and determine the cytokine secretion profile of TRAC CAR T cell. TRAC CAR T cells were also analyzed by flow cytometry to determine the frequency of CD62L and CD45RA population within CD8+ CAR+ T cells (day 0 and day 5 post tumor cell-dependent activation). b Frequency of T cell subpopulation displaying CD62L+CD45RA+ (naive-like), CD62L+ CD45RA− (central memory), CD62L-CD45RA− (effector memory), CD62L-CD45RA+ (terminal effector) labeling and obtained at day 0 and day 5 post tumor cell-dependent activation for different engineered T cells. A linear mixed model, using lmer from the lme4 R package was used for statistical analysis. p-values are documented in Supplementary Table 1 . c Cytokine profiling assay results obtained from supernatant of engineered T cell/RAJI cells cocultured for 5 days. The data shown in b and c represent the average of three experiments performed with cells engineered from three different donors. The mean of cytokine concentration fold change and the whiskers representing the maximum and minimum data points are illustrated in c . Two-way ANOVA was used in panel c for statistical analysis (p-value are indicated on the figures). Source data are provided as a Source Data file Full size image Finally, to assess the influence of tumor cell-dependent IL-12P70 secretion in a more complex system and test the robustness of our in vitro characterization, we evaluated the antitumor activity of TRAC CAR T cells in vivo using a NSG xenograft tumor model (Fig. 8 ). As a proof of concept, we focused on the engineering at the PDCD1 locus rather than the IL2rα locus because (1) concomitant inactivation of PD1 and secretion of IL-12 represents a dual advantage for TRAC CAR T cell functions and bears high potential for clinical application and (2) the PDCD1 locus supported IL-12P70 secretion in smaller amounts than the IL2rα locus in vitro (Fig. 3h , 4b , 6c, and 7c ). Thus, it was of particular interest to test whether the more moderate of the two approaches already has antitumor benefit in vivo. Consistent with earlier results, TRAC CAR _ΔPD1 IL12 was found to control tumor growth better (Fig. 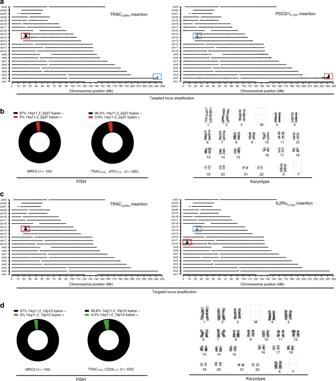Fig. 2 Cytogenetic and genomic characterization of engineered TRACCART cells.aTargeted locus amplification (TLA) analysis of TRACCAR_ΔPD1IL12cells using TRACCARmspecific primers (left panel) or PDCD1IL12mspecific primers (right panel). Specific targeted integration coverages and potential concatemere or homology-independent integrations are indicated by red and blue boxes, respectively.b, left panel Frequency of translocation events between TRAC and PDCD1 loci detected by FISH in MRC5 standard cell line (n= 100 metaphases analyzed) and in TRACCAR_ΔPD1IL12(n= 500 metaphases analyzed). Cells harboring or not the expected gene fusion named 14q11.2_2q37 are illustrated in red or black, respectively and the number of metaphase analyzed for each sample are indicated.b, right panel Representative example of TRACCAR_ΔPD1IL12cells karyotype showing normal ploidy level and no sign of genetic alteraction of TRAC and PDCD1 chromosomal loci.cTargeted locus amplification analysis of TRACCAR_CD25IL12cells using TRACCARmspecific primers (left panel) or IL2rαIL12mspecific primers (right panel). Specific targeted integration coverages and potential concatemere integrations are indicated by red and blue boxes, respectively.d, left panel Frequency of translocation events between TRAC and IL2rα loci detected by FISH in MRC5 standard cell line (n= 100 metaphases analyzed) and in TRACCAR_CD25IL12(n= 500 metaphases analyzed). Cells harboring or not the expected gene fusion named 14q11.2/10p15.1 are indicated in red and black, respectively and the number of metaphase analyzed for each sample are indicated. Chi square was used to calculate the statistical significance of FISH analysis.d, right panel Representative example of TRACCAR_CD25IL12karyotype showing normal ploidy and no sign of genetic alteration of IL2rα and TRAC chromosomal loci. The TLA and FISH plots and Karyotype figures represents 1 experiment performed with 1 donor. Source data are provided as a Source Data file 8b , Supplementary Table 2 ) and to extend mice survival significantly over its TRAC CAR or TRAC CAR _ΔPD1 counterparts (Fig. 8c , p = 0.026 and 0.003, respectively, Log-rank Mantel cox test). This improvement of antitumor activity was not associated with weight loss in the TRAC CAR _ΔPD1 IL12 group within the first 45 days, except for one mouse that died without any sign of tumor relapse 14 days post tumor injection (Supplementary Fig. 8 ). Altogether, our results indicate that the tumor-dependent and regulated expression of IL-12P70 increases the antitumor activity of TRAC CAR T cells and their capacity to accumulate (Fig. 6b ), as well as decreases the frequency of effector memory cells (Fig. 6d, b ) [26] , [53] , recapitulating the known biological and therapeutic benefits of IL-12P70 [8] , [10] , [11] , [51] , [54] , [55] . Fig. 8 Conditional secretion of IL-12P70 increases antitumor activity of TRAC CAR T cells in vivo. a Schematic showing the experimental design to investigate the antitumor activity of engineered TRAC CAR T cells in xenograft mice model. Immunodeficient NSG mice were adoptively transferred on day 0 with RAJI-Luc-GFP tumor cells (2.5 × 10 5 cells per animal in 100 μL of PBS i.v.). Tumor cells were allowed to expand until mice randomization, performed at day 3 on the basis of the level of tumor cell bioluminescence signal. On the same day, mice were adoptively transferred (i.v.) with 7 × 10 6 viable mock-transduced T cells, TRAC CAR T cells ( n = 8), TRAC CAR _ΔPD1 ( n = 8), TRAC CAR _ΔPD1 IL12 ( n = 7) T cells or tumor alone ( n = 4). RAJI-Luc-GFP tumor cell expansion was monitored on various days by bioluminescence imaging (BLI) up to 142 days. b Evolution of average radiance as a function of time for the different mouse cohorts. Dotted lines correspond to the average radiance recorded for individual mouse. Comparison of tumor growth was done using the aucVardiTest function of the clinfun R package. P -value are indicated in the Supplementary Table 2 . c Kaplan Meier plot obtained for different mice cohorts. Log-rank (Mantel-Cox) test was used for statistical analysis ( p -value are indicated on the figures). Source data are provided as a Source Data file Full size image The goal of this work was to engineer smart CAR T cells that are able to sense and react to their environment in a tailored, highly regulated, and antigen-specific manner. As a proof of concept, we simultaneously repurposed TRAC along with the IL2rα or PDCD1 genes to express a CAR at the surface of primary T cells and to harness T cell engagement with tumor cell targets to promote conditional and transient secretion of IL-12P70. Using a combination of TALEN technology and AAV6 embedding promoter-less repair matrices, we efficiently delivered the CAR to the TRAC locus and to target IL-12P70 to the IL2rα and PDCD1 loci. This multiplex targeted insertion led to the disruption of PDCD1 and TRAC genes and to the non-disruptive modification of the IL2rα gene, ultimately allowing the expression of a CAR and the secretion of IL-12P70 in the media. This secretion was transient, dependent on tumor cell engagement, and followed the tight regulation patterns of CD25 and PD1 observed upon T cell activation. The levels of IL-12P70 secreted in the media were sufficient to enhance the short-term and long-term antitumor activity and the capacity of TRAC CAR T cells to accumulate. In addition, our approach prevented the surface expression of PD1, one of the major checkpoints of T cell function. Repurposing of these three genes enabled engineered TRAC CAR T cells to secrete IL-12P70 in a tumor cell-dependent manner without causing commonly reported side effects in vitro [20] . Indeed, the insertion of an IL-12P70 secretion cassette under the control of the NFAT promoter in primary T cells via gammaretroviral transduction has been reported to impair T cell proliferation ex vivo and in vivo [20] , [48] . This lack of proliferation was linked to the gammaretrovirus mediated random insertion of IL-12P70 and to the leakiness of the NFAT-IL-12P70 secretion cassette, even in the absence of a tumor cell target (Supplementary Fig. 6 and ref. [20] ). The targeted insertion of IL-12P70 reported in this study did not impact the viability and proliferation capacity of TRAC CAR T cells and did not lead to unwanted secretion of IL-12P70 in the absence of tumor cells (Fig. 4a, b , Suplementary Figs. 4d–e and 5). In the presence of tumor cells, however, TRAC CAR T cells secreting IL-12P70 accumulated significantly more than their control TRAC CAR T cell counterparts (Fig. 6b , p ≤ 0.0052 for TRAC CAR _CD25 IL12 and TRAC CAR _ΔPD1 IL12 , two-way ANOVA), likely due to IL-12P70 preventing activation cell death [56] . This finding indicates that the IL2rα and PDCD1 regulatory elements and patterns of activation can efficiently prevent unwanted leakiness of IL-12P70 secretion, which can be deleterious for CAR T cell expansion [20] , [57] . Although this targeted insertion strategy avoids the common drawbacks of gammaretrovirus-dependent or lentivirus-dependent random transgene insertions [58] , it may have some downsides. Indeed, although correct targeted matrix insertion occurred in the majority of modified cells without detectable random matrix insertion, a minority of them harbored TRAC CARm insertion at IL2Rα or PDCD1 loci and IL2Rα IL12P70m or PDCD1 IL12P70m insertion at the TRAC locus. These homology-independent integrations were also recently reported after simultaneous editing of TRBC and TRAC loci [34] and a series of different pairs of genes using CRISPR-CAS9 and non-virally delivered template DNA [31] . As demonstrated [31] , these marginal events are unlikely to promote transgene expression because of the lack of exogenous promoter in the matrices and given the potential mismatches between targeted loci and transgenes’ open reading frames. Thus, although this phenomenon warrants a systematical investigation prior to clinical use, we believe that this phenomenon is unlikely to promote aberrant adverse events. To reduce the risks posed by homology-indepent integrations, an alternative may be to separate the engineering of the two loci in time. For example, performing a sequential TALEN treatment would prevent simultaneous double strand-break formation at 2 loci and limit the risk of off-target insertion. This approach could also be beneficial to prevent translocations. To that matter, although accurate quantification of translocation was limited by the low sensitivity of FISH analysis, our results suggest that there is no detectable proliferative advantage conferred by PD1/TRAC translocations during cell expansion. Further work should assess this point before clinical applications. Our work shows that engineered TRAC CAR T cells are able to sense subtle differences in tumor cell concentration and to secrete IL-12P70 accordingly. The level of IL-12P70 secretion correlated with the quantity of tumor cells present in the media in a saturated fashion (Fig. 4b ). In addition, secretion appeared to increase rapidly upon tumor cell engagement and decreased at a rate similar to that observed for tumor disappearance (Figs. 4a and 6a ). Thus, engineered TRAC CAR T cells could be considered as a rheostat that quantitatively and rapidly adapt their IL-12P70 secretion output as a function of tumor cell concentration input. This fine reactivity is likely due to the simultaneous repurposing of TRAC and either IL2rα or PDCD1, which enables successful repuposing of their regulatory elements and recapitulates the natural and exquisite regulation of the TCR pathway. Therefore, our work shows that it is possible to modify interconnected genetic elements to rewire the cellular circuitry and transform biological inputs into relevant therapeutic outputs. The low and transient levels of IL-12P70 secreted by engineered TRAC CAR T cell were sufficient to elicit greater antitumor activity than control TRAC CAR T cells in vitro and in vivo. The activation-induced secretion of IL-12p70 also correlated with a increased level of IL-2, TNFα, IL-10 and cell surface presentation of CD62L, a marker expressed in the central memory, stem memory, and naive T cells. This phenotype was previously reported for T cells activated in the presence of IL-12P70 [11] , [50] , [51] , [52] . These positive effects are likely to be enhanced in vivo by the ability of IL-12P70 to recruit innate immune cells, which synergistically improve CAR T cell antitumor activity [10] , [59] . This particular aspect should be further investigated in an immunocompetent mouse model. Engineering CAR T cells with customized therapeutic response programs was first reported using single therapeutic transgenes under the control of generic exogenous promoters. However, the constitutive nature of transgene expression under these conditions and the potential toxicity associated with these engineering strategies led to the development of inducible expression systems that take advantage of drug-inducible or tumor-inducible promoters and, more recently, to the engineering of synthetic Notch receptors [48] , [60] , [61] , [62] , [63] . Here we chose a different approach that takes advantage of the highly regulated nature of immune pathways to endow CAR T cells with customized activity. The precise repurposing of endogenous genes reported in this work allows users to bypass the need for an exogenous promoter and exploits optimized regulatory networks to express a therapeutic transgene of interest in a conditional fashion. More importantly, thanks to the availability of high content databases reporting temporal gene transcription and protein expression in various physiological environments [64] , [65] , one can customize the amplitude and kinetics of therapeutic transgene delivery by choosing the gene to rewire in a strategic manner. Endogenous gene network repurposing becomes now possible with the recent advances of gene editing technics [66] and DNA template vectorization methods (single and double DNA templates [31] , [34] , [67] , [68] , [69] , and AAV6-embeded template [26] , [29] , [32] , [70] ). Our work illustrates the therapeutic potential of this approach by rewiring different elements of the TCR activation pathway, but is not limited to it. Indeed, it can be extended to other gene networks to sense a wide variety of relevant inputs (e.g., tumor microenvironment biomarkers such as acidosis, oxygen, and arginine deprivation) and to translate them into different genetically encoded therapeutic outputs. Thus, our work paves the way for the repurposing of genetic pathways to generate smart CAR T cells that are able to integrate complex environmental inputs and to generate custom outputs in a highly regulated and specific manner. Biological materials Cryopreserved human PBMCs were acquired from ALLCELLS (cat # PB006F) and used in accordance with Cellectis IRB/IEC-approved protocols. PBMCs were cultured in X-vivo-15 media (obtained from Lonza Group, cat # BE04-418Q), containing IL-2 (obtained from Miltenyi Biotech, cat # 130-097-748), and human serum AB (obtained from Seralab, cat # GEM-100-318). Human T activator CD3/CD28 from Life Technologies/Thermo Fisher Scientific (cat # 11132D) was used to activate T cells. TRAC CAR T cells were purified using a CD34 MicroBead kit and a MACS® LD-column from Miltenyi Biotech (cat # 130-046-702 and cat # 130-042-901, respectively). Post-staining was carried out with antibody QBEND10-APC from R&D Systems (cat # FAB7227A). All other antibodies used and the corresponding concentrations are summarized in Table 1 . Table 1 Antibodies used in the study Full size table Targeted integration of CAR and IL-12P70 constructs The double targeted integration at the TRAC and PDCD1 or IL2rα loci were performed as follows: PBMC cells were thawed, washed, resuspended, and cultivated in X-vivo-15 complete media (X-vivo-15, 5% AB serum, 20 ng/mL IL-2). One day later, the cells were activated with Dynabeads human T activator CD3/CD28 (25 µL of beads/10 6 CD3 positive cells) and cultivated at a density of 10 6 cells/mL for 3 days in X-vivo complete media at 37 °C in the presence of 5% CO 2 . The cells were then split into fresh complete media and transduced/transfected the next day according to the following procedure. On the day of transduction-transfection, the cells were first de-beaded by magnetic separation (EasySep), washed twice in Cytoporation buffer T (BTX Harvard Apparatus, Holliston, Massachusetts), and resuspended at a final concentration of 28E 6 cells/mL in the same solution. This cellular suspension was mixed with 5 µg mRNA encoding TRAC TALEN arms in the presence or absence of 15 µg of mRNA encoding arms of either PDCD1 or IL2rα TALEN (please refer to Supplementary Data 2 for the TALEN arm mRNA sequences and Table 2 for the target DNA sequences) in a final volume of 200 µl. Transfection was performed using Pulse Agile technology by applying two 0.1 mS pulses at 3000 V/cm followed by four 0.2 mS pulses at 325 V/cm in 0.4 cm gap cuvettes and in a final volume of 200 µL of Cytoporation buffer T (BTX Harvard Apparatus, Holliston, Massachusetts). The electroporated cells were then immediately transferred to a 12-well plate containing 1 mL of prewarmed X-vivo-15 serum-free media and incubated at 37 °C for 15 min The cells were then concentrated to 8E 6 cells/mL in 250 µL of the same media in the presence of AAV6 particles (MOI = 3E 5 vg/cells) comprising the donor matrices (Supplementary Data 1 ) in 48-well regular treated plates. After 2 h of culture at 30 °C, 250 µL of Xvivo-15 media supplemented by 10% AB serum and 40 ng/mL IL-2 was added to the cell suspension, and the mix was incubated for 24 h under the same culture conditions. One day later, the cells were seeded at a density of 10 6 cells/mL in complete X-vivo-15 media and cultivated at 37 °C in the presence of 5% CO 2 . Table 2 TALEN targets used in the study Full size table Lentivirus-based engineering of T cells PBMC cells were thawed, washed, resuspended, and cultivated in X-vivo-15 complete media (X-vivo-15, 5% AB serum, 20 ng/mL IL-2). One day later, the cells were activated with Dynabeads human T activator CD3/CD28 (25 µL of beads/10 6 CD3 positive cells) and cultivated at a density of 10 6 cells/mL for 3 days in X-vivo complete media at 37 °C in the presence of 5% CO 2 . The cells were incubated on retronectin coated plates, with 2 independent lentiviral particles encoding CD22 CubiCAR (MOI 5) and IL-12P70 under the control of 6 NFAT promoter followed by a minimal IL-2 promoter (MOI 0.25 [20] , [48] ) in Xvivo-15 media and were supplemented by 1 volume of Xvivo 10% Ab serum, 40 ng/mL IL-2 and incubated overnight. One day later, cells were seeded at a density of 10 6 cells/mL in complete X-vivo-15 media and cultivated at 37 °C in the presence of 5% CO 2 . Isolation of TRAC CAR T cells using magnetic separation TRAC CAR T cells were purified 4 days after transduction using a CD34 MicroBead kit and MACS-LD column from Miltenyi Biotech as previously described [36] . Briefly, 5–10 × 10 7 T cells were incubated with 100 µL of FC-blocking reagent and 125 µL QBEND10 coated magnetic beads for 30 min in a final volume of 500 µL CliniMACS Buffer. The cellular suspension was then loaded onto a MACS® LD-Column attached to a conventional Myltenyi magnet and washed three times with 1 mL of CliniMACS Buffer. The column was eventually removed from the magnet, and the TRAC CAR T cells were eluted in 3 mL of the same buffer. One round of purification was sufficient to obtain a homogeneous population of CubiCAR T cells (purity > 96%). Cytogenic characterization of TRAC CAR T cells Engineered TRAC CAR T cells expanded for a total of 17 days in G-Rex were subjected to TLA, FISH, and karytope analysis. Karyotype and fluorscence in situ hybridization (FISH) TRAC CAR T cells were incubated with RAJI cells (E/T ratio = 1) for 3 days to allow them to divide. Dividing TRAC CAR T cell were then fixed and hybridized with TRAC, PDCD1, or IL2Rα specific fluorescent probes according to FISH standard procedures ( Supplementary Materials section ). The same procedure was performed with MRC-5, a human fibroblast cell line considered as a reference diploid cell line by the European Medicine Agency and commonly used as a negative control for gene fusion detection by FISH. 100 metaphasic nuclei from the MRC-5 negative control and 500 metaphasic nuclei from TRAC CAR T cells were screened for fusions of the TRAC gene (14q11.2) with either the PDCD1 gene (2q37.3) or IL2Rα gene (10p15.1). Regarding Karyotype, a total of one hundred metaphases were studied for each sample. Eighty (80) metaphases were screened for aberrations of the TRAC and PDCD1 chromosomal loci (14q11.2 and 2q37) or TRAC and IL2Rα chromosomal loci (14q11.2 and 10p15.1), the ploidy level (hyperploidy, hypoploidy, polyploidy) and the modal chromosome number determination but also, for any gross structural abnormalities including chromosome breaks and gaps among others (dicentrics, acentric fragments). Twenty additional metaphases were karyotyped according to the International System for Chromosome Nomenclature (ISCN) based on their G-banding pattern for the detection of any specific structural chromosomal aberration including deletions, translocations involving 14q11.2/2q37 or 14q11.2/10p15.1, inversions, duplications and additions. The modal chromosome number of the 2 tested samples, originating from the same T cell donor, was defined as 46 chromosomes (22 pairs of autosomes and one pair of sex chromosomes) and the sex of the sample was female. Experiments were performed by Cleancells (Bouffere, Frnace). Targeted locus amplification (TLA) TLA analysis of engineered TRAC CAR T cell was performed by Cergentis (Utrecht, Netherlands) according to ref. [40] using a set of multiple primers described in Supplementary Tables 3 – 4 . 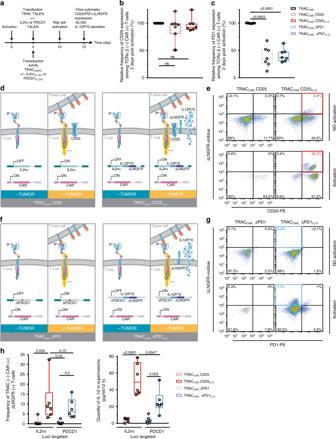Fig. 3 Efficient translation of tumor cell engagement by TRACCART cell into IL-12P70 secretion in vitro.aSchematic showing the experimental design used to determine the levels of CD25 and PD1 expression and IL-12P70 secretion by tumor cell-activated TRACCART cells.bandcFrequency of CD25 and PD1 expression detected among TCRαβ (−) and CAR (+) T cells, respectively. Each point represents one experiment performed with a given donor (n= 7). One-way ANOVA was used in panel3band3cfor statistical analysis andp-value are indicated.dSchematic showing the expected outcome of IL-12P70 secretion upon tumor cell engagement by TRACCAR_CD25 or TRACCAR_CD25IL12T cells.eFlow cytometry plots showing ΔLNGFR surface expression 48 h after tumor cell-dependent activation of TRACCAR_CD25 and TRACCAR_CD25IL12T cells. The flow plot was obtained using engineered TRACCART cell batches harboring the highest IL-12P70 targeted integration. The red box indicates the proportion of ∆LNGFR expressed by successfully engineered TRACCART cells. Gating strategy is illustrated in Supplementary Fig.4.fSchematic showing IL-12P70 secretion upon tumor cell engagement by TRACCAR_ΔPD1 or TRACCAR_ΔPD1IL12T cells.gFlow cytometry plots showing the level of ΔLNGFR expression, 48 h after tumor cell-dependent activation of TRACCAR_CD25 and TRACCAR_CD25IL12T cells. The solid blue squares indicate the frequency of ∆LNGFR expression by successfully engineered TRACCART cells. Gating strategy is illustrated in Supplementary Fig.4.hFrequency of ∆LNGFR expression (left panel) and quantity of IL-12P70 secreted (right panel) by TRACCART cells engineered at the IL2rα and PDCD1 loci, 48 h after tumor cell-dependent activation of the TRACCART cells. Each point represents one experiment performed with a given donor (n= 6) and the threshold of IL-12P70 detection is 5 pg/mL. On each box plot, the central mark indicates the median, the bottom and top edges of the box indicate the interquartile range (IQR) and the whiskers represent the maximum and minimum data point. One-way ANOVA was used in panel3hfor statistical analysis andp-value are indicated. Source data are provided as a Source Data file Regarding TRAC CAR _ΔPD1 IL12 analysis, 2 primer sets were designed on the genome in the TRAC and PDCD1 loci (Supplementary Table 3 , sets 1–4), and 2 primer sets were designed on TRAC CARm and PDCD1 IL12m , Supplementary Table 3 , sets 5–8). 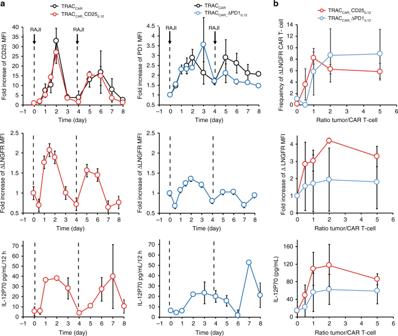Fig. 4 The secretion of IL-12P70 by TRACCART cells is regulated by tumor cell engagement in vitro.aKinetics of CD25 and PD1 expression (top), ΔLNGFR expression (middle), and IL-12P70 secretion (bottom panel) in purified TRACCART cells after two consecutive tumor cells challenges. TRACCART cells were activated by RAJI cells at day 0 and day 4 and analyzed by flow cytometry for 8 days. IL-12P70 secreted in cell culture supernatants was quantified by ELISA and plotted as a function of time. The arrows indicate the times of tumor cell addition. The data shown represent the average +/− standard deviation of two experiments performed with cells from two different donors.bChanges in ΔLNGFR reporter expression and IL-12P70 secretion as a function of tumor cell concentration. Engineered TRACCART cells were activated by different quantities of RAJI cells for 48 h. Supernatants were used to quantify IL-12P70 via ELISA assays and cells were analyzed by flow cytometry to evaluate the frequency of ΔLNGFR+ cells, as well as its mean fluorescence intensity. Values are plotted as a function of the tumor cell to TRACCART cell ratio. The data shown are the average +/− standard deviation of three experiments performed with cells from three different donors. Source data are provided as a Source Data file Regarding TRAC CAR _CD25 IL12 analysis, 2 primer sets were designed on the genome in the TRAC and IL2Rα loci (Supplementary Table 4 , sets 1–4), and 2 primer sets were designed on TRAC CARm and IL2Rα IL12m , 2 sets per matrix (Supplementary Table 4 , sets 5–8). The primer sets were used in individual TLA amplifications. PCR products were purified and library prepped using the Illumina Nextera flex protocol and sequenced on an Illumina sequencer. Reads were mapped using BWA-SW, version 0.7.15-r1140, settings bwasw -b 7. The NGS reads were aligned to the matrices sequence and host genome. The human hg19 genome was used as host reference genome sequence. Integration sites were detected based on a coverage peaks in the genome and on the identification of fusion-reads between the matrices sequence and the host genome. Oligo capture assay To explore the specificity of TALEN targeting, an Oligo capture assay (OCA) derived from ref. [43] was used. The Oligo capture assay detected the on-target and off-target site of TALEN through the incorporation of small duplex oligodeoxynucleotides (dsODNs) into the double-stranded breaks (DSBs) induced by the TALEN nuclease activity. These labeled DSBs were then mapped at nucleotide resolution by amplification of sequences bearing an integrated dsODN and high throughput DNA sequencing. In brief, cells were transfected with TRAC and PDCD1 TALEN and dsODN and propagated for about 6 days. Genomic DNA was harvested from these cells, randomly sheared with a sonicator and end-repaired/A-tailed. Next-generation sequencing Y-adapters (TruSeq Annealed Adapter) that contain the P5 sequence were ligated to the ends of this DNA. Nested, anchored PCR using dsODN-specific and adapter-specific primers were used to specifically amplify the plus and minus strand of DNA fragments that incorporated the dsODN. 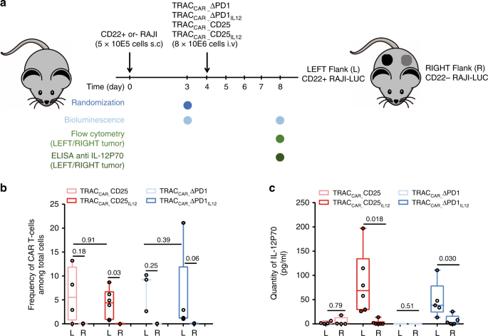Fig. 5 In vivo local and tumor-dependent delivery of IL-12P70 by TRACCART cells.aSchematic showing the experimental design to study the tumor-dependent secretion of IL-12P70 by TRACCART cells in NSG mice (BLI: bioluminescence). CD22(+) and CD22(−) RAJI tumor cells expressing firefly luciferase were transferred subcutaneously into the left (L) and right (R) flanks of NSG mice, respectively, and allowed to engraft for 4 days before TRACCART cell transfer. Four days after TRACCART cells transfer, tumors and T cells were recovered, dissociated, and analyzed via flow cytometry and ELISA.bFrequency of TRACCART cells detected by flow cytometry at the left (L) and right (R) flanks of NSG mice. A non parametric paired Mann-Whitney test was used for statistical analysis of the data (p-value are indicated).cQuantity of IL-12P70 detected in the left (L) and right (R) flanks of NSG mice. Each point documented inbandcrepresents the result obtained in each mice (n= 4 for TRACCAR_CD25,n= 6 for TRACCAR_CD25IL12,n= 3 for TRACCAR_ΔPD1,n= 5 for TRACCAR_ΔPD1IL12). On each box plot, the central mark indicates the median, the bottom and top edges of the box indicate the interquartile range (IQR) and the whiskers represent the maximum and minimum data point. A paired Wilcoxon-Mann-Whitney non-parametric test was used for statistical analysis of the IL-12P70 quantities obtained at the right and left flanks of the same animal (p-value are indicated). Source data are provided as a Source Data file The first round of PCR used the following adapter-specific (P5_1) and dsODN-specific primers. The second round of PCR used the following adapter-specific (P5_2) and dsODN-specific primers along with a third oligo P7 that added the barcode and P7 sequence to the ends of the DNA. Equal amounts of these separate PCRs were pooled together and sequenced using Illumina MiSeq (2 × 150 bp). The resulting sequences were then mapped on human genome to identify potential offsite candidate. Potential off-site candidate identified by OCA were then verified using genomic DNA obtained from T cells transfected by PDCD1 and TRAC in the absence of dsODN. Genomic DNA was amplified using off-site candidate-specific PCR primer pairs and the resulting amplicons were analyzed by high throughput DNA sequencing to determine the frequency of Indels genetrated the TALEN treatment. Activation-dependent expression of ΔLNGFR and IL-12P70 Engineered TRAC CAR T cells were recovered from the transfection-transduction process described above and seeded at 10 6 cells/mL alone or in the presence of RAJI tumor cells (Effector: target, E:T = 1:1) in a final volume of 100 µL of X-vivo-15 media supplemented with 5% AB serum. Cells were collected every day for 8 days after activation, labeled, and analyzed by flow cytometry using specific antibodies. From the same experimental set up, 100 µL of supernatant was collected each day to measure IL-12P70 secretion in the media using an IL-12P70 specific ELISA kit by R&D systems according to the manufacturer’s protocol. Serial killing assay To assess the antitumor activity of engineered TRAC CAR T cells, a serial killing assay was performed using a protocol similar to that reported in [36] . TRAC CAR T cells were mixed with a suspension of 2 × 10 5 RAJI-luc tumor cells at E:T = 5:1 in a total volume of 1 mL of Xvivo-15 media supplemented with 5% AB serum. The mixture was incubated for 24 h before determining the luminescence of 25 µL of cell suspension using 25 µL of ONE-Glo reagent (Promega). 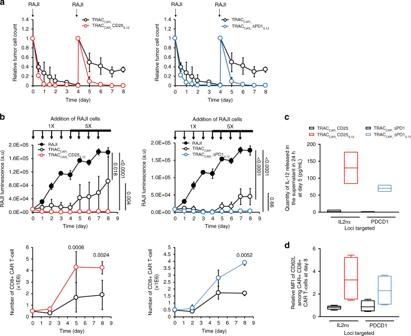Fig. 6 Conditional secretion of IL-12P70 increases TRACCART cells antitumor activity in vitro.aKinetics of tumor cell clearance by purified TRACCART cells and TRACCART cells secreting IL-12P70. TRACCAR, TRACCAR_CD25IL12T cells and TRACCAR_ΔPD1IL12T cells were challenged with 1 equivalent of RAJI cells at days 0 and 4 and cultivated for 8 days. Kinetics of tumor cell disappearance was analyzed by integrating flow cytometry data, using CD19 antibody specific for RAJI cells, and total number of cells mixture. The relative tumor cell count was computed as the ratio of remaining tumor cells at a given time to the total number of tumor cells added.bLong-term cytotoxicity assay. TRACCART cells were challenged daily with RAJI cells at a ratio of T cells to tumor cells of 5-to-1. Fresh tumor cells (0.2 × 106cells) were added everyday up to day 4 after pelleting and resuspended the TRACCART cells in fresh culture media. From day 5 onward, 5× the original number of tumor cells (106cells) was added. The antitumor activity of the TRACCART cells was monitored everyday by measuring the luminescence of the remaining RAJI tumor cells expressing luciferase. Cells were counted and analyzed by flow cytometry on days 0, 2, 5, and 8, and the number of CD8 (+) CAR T cells was computed and plotted as a function of time. The data are averaged +/− standard deviation from two experiments performed with cells from two different donors. Two-way ANOVA was used in panelbfor statistical analysis (p-value are indicated).cComparison of IL-12P70 secretion for different TRACCART cell groups at day 5 of the serial killing assay.dComparison of CD62L MFI among CD8 (+) CAR T cells obtained for the different TRACCART cell groups at day 8 of the serial killing assay. The data shown incanddwere obtained from two experiments performed with cells from two different donors. On each box plot, the central mark indicates the median, the bottom and top edges of the box indicate the interquartile range and the whiskers represent the maximum and minimum data point. Source data are provided as a Source Data file The cell mixture was then spun down, and the old media was discarded and substituted with 1 mL of fresh complete Xvivo-15 media containing 2 × 10 5 RAJI-Luc cells. The resulting cell mixture was incubated for 24 h. This protocol was repeated up to 4 days. The same protocol was used from days 5 to 8 with the daily addition of 5 times more RAJI-Luc cells. A similar protocol was used to investigate the effector and memory phenotype and cytokine secretion profile of activated engineered TRAC CAR T cells. 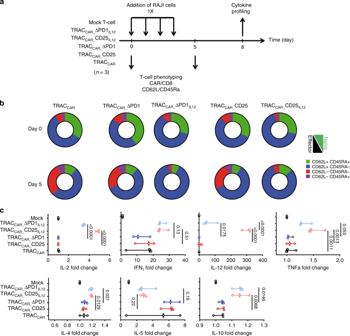Fig. 7 Immunoprofiling of engineered TRACCART cells activated by tumor cells in vitro.aSchematic showing the experimental design to investigate the effector and memory phenotype and cytokine secretion profile of activated engineered TRACCART cells. 106TRACCART cells were mixed with a suspension of RAJI-luc tumor cells at E:T = 5:1 in a total volume of 40 mL of Xvivo-15 media supplemented with 5% AB serum and incubated in a GREX-10 device. The mixture was incubated for 24 h before adding 2 × 106RAJI-Luc cells. The resulting cell mixture was incubated for 24 h and the same procedure was repeated to get a total of 4 RAJI cell challenges. The mixture was then incubated as is for 4 additional days and where spun down to recover the supernatant and determine the cytokine secretion profile of TRACCART cell. TRACCART cells were also analyzed by flow cytometry to determine the frequency of CD62L and CD45RA population within CD8+ CAR+ T cells (day 0 and day 5 post tumor cell-dependent activation).bFrequency of T cell subpopulation displaying CD62L+CD45RA+ (naive-like), CD62L+ CD45RA− (central memory), CD62L-CD45RA− (effector memory), CD62L-CD45RA+ (terminal effector) labeling and obtained at day 0 and day 5 post tumor cell-dependent activation for different engineered T cells. A linear mixed model, using lmer from the lme4 R package was used for statistical analysis. p-values are documented in Supplementary Table1.cCytokine profiling assay results obtained from supernatant of engineered T cell/RAJI cells cocultured for 5 days. The data shown inbandcrepresent the average of three experiments performed with cells engineered from three different donors. The mean of cytokine concentration fold change and the whiskers representing the maximum and minimum data points are illustrated inc. Two-way ANOVA was used in panelcfor statistical analysis (p-value are indicated on the figures). Source data are provided as a Source Data file 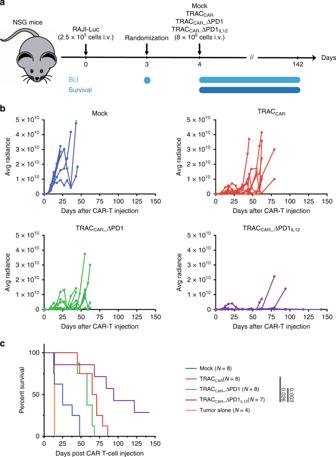Fig. 8 Conditional secretion of IL-12P70 increases antitumor activity of TRACCART cells in vivo.aSchematic showing the experimental design to investigate the antitumor activity of engineered TRACCART cells in xenograft mice model. Immunodeficient NSG mice were adoptively transferred on day 0 with RAJI-Luc-GFP tumor cells (2.5 × 105cells per animal in 100 μL of PBS i.v.). Tumor cells were allowed to expand until mice randomization, performed at day 3 on the basis of the level of tumor cell bioluminescence signal. On the same day, mice were adoptively transferred (i.v.) with 7 × 106viable mock-transduced T cells, TRACCART cells (n= 8), TRACCAR_ΔPD1 (n= 8), TRACCAR_ΔPD1IL12(n= 7) T cells or tumor alone (n= 4). RAJI-Luc-GFP tumor cell expansion was monitored on various days by bioluminescence imaging (BLI) up to 142 days.bEvolution of average radiance as a function of time for the different mouse cohorts. Dotted lines correspond to the average radiance recorded for individual mouse. Comparison of tumor growth was done using the aucVardiTest function of the clinfun R package.P-value are indicated in the Supplementary Table2.cKaplan Meier plot obtained for different mice cohorts. Log-rank (Mantel-Cox) test was used for statistical analysis (p-value are indicated on the figures). Source data are provided as a Source Data file 10 6 TRAC CAR T cells were mixed with a suspension of RAJI-luc tumor cells at E:T = 5:1 in a total volume of 40 mL of Xvivo-15 media supplemented with 5% AB serum and incubated in a GREX-10 device. The mixture was incubated for 24 h before adding 2 × 10 6 RAJI-Luc cells. The resulting cell mixture was incubated for 24 h and the same procedure was repeated to get a total of 4 RAJI cell challenges. The mixture was then incubated as is for 4 additional days and where spun down to recover the supernatant and determine the cytokine secretion profile of TRAC CAR T cell. TRAC CAR T cells were also analyzed by flow cytometry to determine the frequency of CD62L and CD45RA population with CD8+ CAR + T cells (at day 0 and 5 post activation). In vivo experiment using NGS xenograft model All procedures involving animals were performed in accordance with regulations and established guidelines and were reviewed and approved by the Cellectis Institutional Animal Care and Use Committee (IACUC), as well as by the Animal Ethical Committee at Mispro-Biotech (New York, NY). Tumor-dependent secretion of IL-12P70 in vivo A total of 40 immunodeficient NSG mice (NOD.Cg- Prkdc scid Il2rg tm1Wjl /SzJ, the Jackson Laboratory), were received and acclimatized for a week. NSG mice were then injected with 0.5 × 10 6 CD22+ RAJI and CD22− RAJI tumor cells on left and right flank, respectively. The tumor cells were allowed to expand until mouse randomization, which was performed at day 4 based on the degree of tumor cell outgrowth, measured using bioluminescence imaging (BLI) (XenoLight D-luciferin (PerkinElmer). The next day, mice were adoptively transferred (i.v.) with either 8 × 10 6 viable mock-transduced T cell or 8 × 10 6 viable TRAC CAR positive T cells (7 mice per group, total 5 groups). The mice were then re-imaged at day 6 of TRAC CAR T cell injection and sacrificed to harvest serum, spleen, and right and left tumors. The splenocytes were prepared by mechanical disruption of the organ followed by 70 µm-filtering and a Ficoll density gradient purification. The cell suspensions were analyzed by flow cytometry. The tumors were dissociated using Miltenyi’s human tumor dissociation buffer according to the manufacturer’s protocol. The cells were then filtered using a 40 µm filter and analyzed by flow cytometry. Antitumor activity of TRAC CAR T cell in vivo A total of 35 immunodeficient NSG (NOD.Cg- Prkdc scid Il2rg tm1Wjl /SzJ, the Jackson Laboratory) mice were adoptively transferred on day 0 with RAJI-Luc-GFP tumor cells (2.5 × 10 5 cells per animal in 100 μL of PBS i.v.). Tumor cells were allowed to expand until mice randomization, performed at day 3 on the basis of the level of tumor cell bioluminescence signal . On the same day, mice were adoptively transferred (i.v.) with 7 × 10 6 viable Mock-transduced T cells, TRAC CAR T cells, TRAC CAR _ΔPD1, TRAC CAR _ΔPD1 IL12 T cells or no T cells. This amount of cells correspond to the actual CAR positive cell numbers injected. The different group were constituted by 8 mice for except TRAC CAR _ΔPD1 IL12 T cells ( N = 7) and tumor alone group ( N = 4). RAJI-Luc-GFP tumor cell expansion was monitored on various days by bioluminescence imaging (BLI) using XenoLight D-luciferin (PerkinElmer), injected i.p. in animals (150 μL, 10 mg/mL stock solution) before induction of narcosis (isoflurane). Data acquisition and was performed 5 min Xenolight D-luciferine injection using a Spectrum-CT apparatus (Perkin Elmer) interfaced to Living Image software (Caliper). Average Radiance was determined and plotted as a function of time to reflect tumor growth curve.